Activation of TRPC6 channels is essential for lung ischaemia–reperfusion induced oedema in mice Lung ischaemia–reperfusion-induced oedema (LIRE) is a life-threatening condition that causes pulmonary oedema induced by endothelial dysfunction. Here we show that lungs from mice lacking nicotinamide adenine dinucleotide phosphate (NADPH) oxidase ( Nox2 y/− ) or the classical transient receptor potential channel 6 ( TRPC6 −/− ) are protected from LIR-induced oedema (LIRE). Generation of chimeric mice by bone marrow cell transplantation and endothelial-specific Nox2 deletion showed that endothelial Nox2, but not leukocytic Nox2 or TRPC6, are responsible for LIRE. Lung endothelial cells from Nox2- or TRPC6-deficient mice showed attenuated ischaemia-induced Ca 2+ influx, cellular shape changes and impaired barrier function. Production of reactive oxygen species was completely abolished in Nox2 y/− cells. A novel mechanistic model comprising endothelial Nox2-derived production of superoxide, activation of phospholipase C-γ, inhibition of diacylglycerol (DAG) kinase, DAG-mediated activation of TRPC6 and ensuing LIRE is supported by pharmacological and molecular evidence. This mechanism highlights novel pharmacological targets for the treatment of LIRE. Lung ischaemia–reperfusion oedema (LIRE) is one of the most common and significant causes of morbidity and mortality after lung transplantation, thrombarterectomy and acute lung embolism [1] . LIRE typically results in massive damage of the microvascular endothelium, lung oedema and consequent organ dysfunction, and despite considerable progress in the management of this disorder, the molecular mechanism underlying its development remains unclear [1] . Early during LIRE, there is a rise in reactive oxygen species (ROS) [2] and intracellular Ca 2+ concentration ([Ca 2+ ] i ) in endothelial cells [3] . This has been proposed to be an initial step in the pathogenesis of injury, which would then lead to a change in cell morphology and increased endothelial permeability [4] , [5] , followed by the subsequent extravasation of plasma, macromolecules and immune cells. However, the contribution of different cell types to this process and the underlying signalling cascade are still elusive. In particular, the question of how ROS production and endothelial [Ca 2+ ] i is regulated in LIRE has not yet been answered. Although a 'burst' of ROS during LIRE has been observed by many investigators [2] , the major source of ROS production remains unclear. One likely candidate is the nicotinamide adenine dinucleotide phosphate (NADPH)-dependent oxidase that is present in the plasma membrane of the polymorphonuclear (PMN) leukocytes [6] and contains six subunits: rac1 or rac2 and five phox proteins. The catalytic core of the enzyme is located in the Nox2 protein (also known as gp91 phox ), which also contains the heme molecule [6] . Although a deleterious role for circulating PMN leukocytes in LIRE has been inferred from the protective effect of depletion of PMN leukocytes [7] and from the reduction in injury following inhibition of adhesion molecules [8] , the role of resident lung leukocytes in LIRE remains controversial [9] , [10] , [11] . In addition to leukocytes, a phagocyte-type NADPH oxidase expressed in endothelial cells is a major contributor to the overall vascular ROS production and has a key role in vascular oxidative stress [12] . Although ROS derived from vascular NADPH oxidase have been implicated in the pathophysiology of many cardiovascular diseases, including atherosclerosis, hypertension, diabetic vasculopathy and heart failure, their role in LIRE remains undefined. Transient receptor potential (TRP) channels are regulators of [Ca 2+ ] i in many tissues, including vascular smooth muscle and endothelium, and may be crucial contributors to the rise in endothelial [Ca 2+ ] i during LIRE. The TRP protein superfamily consists of a diverse group of non-selective cation channels involved in many basic cellular processes [13] . Although the members of the TRPV (for vanilloid) and TRPM (for melastatin) subfamilies have emerged as versatile cellular sensors, the functional importance of the seven members of the TRPC (for classical) channel subfamily (TRPC1–7) is still poorly understood [13] . Among the TRPC channels, TRPC3, 6 and 7 share 69% identity and are gated by pathways involving C-type phospholipases (PLCs) and by direct exposure to diacylglycerols (DAG) [14] . TRPC6 is highly expressed in the lung, and we recently demonstrated that it has an essential role during acute hypoxic vasoconstriction [15] . Recent studies have demonstrated that TRPC6 represents a target of ROS in different disease models [16] , [17] , [18] , [19] . Furthermore, there is evidence that TRPC6 is involved in thrombin-induced Ca 2+ entry into endothelial cells and a subsequent change of cell shape [20] . Therefore, our data propose a mechanistic model in which ROS production by activated endothelial NOX2 leads to PLCγ activation, DAG kinase inhibition and subsequent TRPC6 activation as successive events resulting in LIRE. Nox2 and TRPC6 induce vascular permeability after reperfusion To address the importance of Nox2 in LIR-induced oedema (LIRE), we analysed isolated lungs from wild-type (WT) and Nox2-deficient ( Nox2 y/− ) mice [21] ( Supplementary Methods ). After 90 min of ischaemia and application of three hydrostatic challenge manoeuvres at 30, 60 and 90 min after reperfusion, WT lungs showed enhanced vascular permeability, as evidenced by a considerable gain in lung weight ( Fig. 1a ) and an increased capillary filtration coefficient (Kfc) ( Fig. 1b ). By contrast, lungs isolated from Nox2 y / − mice were almost completely protected from ischaemia–reperfusion-induced increase in organ weight ( Fig. 1a ) and in Kfc values ( Fig. 1b ). In non-ischaemic lungs, Kfc values were essentially constant and only marginal lung weight gains were observed throughout the entire experimental period ( Fig. 1a,b ). The NADPH oxidase inhibitor and antioxidant apocynin significantly attenuated vascular leakage and reduced lung oedema after ischaemia–reperfusion, similarly to Nox2 deficiency ( Fig. 1a,b ). In contrast, mice deficient in Nox1 or Nox4 were not protected from LIRE, but showed lung weight gain ( Supplementary Fig. S1a ) and increased Kfcs ( Supplementary Fig. S1b ), similar to WT mice. 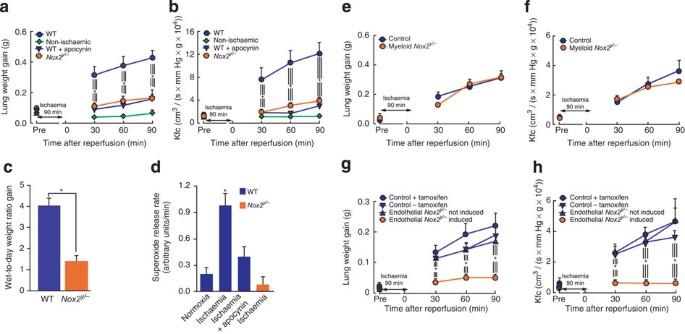Figure 1: Analysis of LIRE in WT and Nox2-deficient lungs, as well as in mice with deficiency for Nox2 in either cells of the myeloid lineage or in endothelial cells. (a,bande–h) Post-ischaemic vascular leakage in isolated lungs. (a,e,g) Lung weight gain was calculated as the weight difference before and after each hydrostatic challenge manoeuvre. (b,f,h) The lung Kfc was determined before ischaemia and at 30-min intervals after re-establishing perfusion. (c) Analysis of ischaemia–reperfusion-induced pulmonary oedema formation in living mice. Pulmonary oedema formation was analysed by quantitative assessment of wet-to-dry weight ratios of ischaemia-exposed lungs, normalized to sham-operated mice. (d) Intravascular superoxide release in isolated lungs±apocynin. (e–h) Myeloid Nox2y/−(=Nox2-flox-flox-LysmCre-+/0) were compared with Nox2-flox-flox-LysmCre-0/0 mice as controls. Endothelial Nox2y/−(=Nox2-flox-flox-ERT2-Tie2-+/0) was compared with Nox2-flox-flox-ERT2-Tie2-0/0 as controls. Values from each mouse line with or without tamoxifen induction are indicated. (a,bande–h)n=4–6. Data were statistically analysed by Student'st-test with Welsh's correction for comparisons of two groups and one-way analysis of variance with the Student–Newman–Keuls test for multiple comparisons. All data are presented as mean±s.e.m.; *P<0.05. For (d) *indicates significant differences compared with 'Normoxia'. Figure 1: Analysis of LIRE in WT and Nox2-deficient lungs, as well as in mice with deficiency for Nox2 in either cells of the myeloid lineage or in endothelial cells. ( a , b and e – h ) Post-ischaemic vascular leakage in isolated lungs. ( a , e , g ) Lung weight gain was calculated as the weight difference before and after each hydrostatic challenge manoeuvre. ( b , f , h ) The lung Kfc was determined before ischaemia and at 30-min intervals after re-establishing perfusion. ( c ) Analysis of ischaemia–reperfusion-induced pulmonary oedema formation in living mice. Pulmonary oedema formation was analysed by quantitative assessment of wet-to-dry weight ratios of ischaemia-exposed lungs, normalized to sham-operated mice. ( d ) Intravascular superoxide release in isolated lungs±apocynin. ( e – h ) Myeloid Nox2 y/− (=Nox2-flox-flox-LysmCre-+/0) were compared with Nox2-flox-flox-LysmCre-0/0 mice as controls. Endothelial Nox2 y/− (=Nox2-flox-flox-ERT2-Tie2-+/0) was compared with Nox2-flox-flox-ERT2-Tie2-0/0 as controls. Values from each mouse line with or without tamoxifen induction are indicated. ( a , b and e – h ) n =4–6. Data were statistically analysed by Student's t -test with Welsh's correction for comparisons of two groups and one-way analysis of variance with the Student–Newman–Keuls test for multiple comparisons. All data are presented as mean±s.e.m. ; * P <0.05. For ( d ) *indicates significant differences compared with 'Normoxia'. Full size image We next investigated lung oedema formation in vivo , in intact anaesthetized mice during ischaemia–reperfusion. Although WT mice developed severe oedema, Nox2 y/− mice did not ( Fig. 1c ). Moreover, total intravascular superoxide release following ischaemia–reperfusion was increased in lungs from WT mice compared with lungs from time-matched non-ischaemic controls ( Fig. 1d ). By contrast, intravascular superoxide release after ischaemia–reperfusion was reduced in lungs from apocynin-treated mice or Nox2 y/− mice compared with those from WT mice. The cellular sources of the different mediators that are suggested to contribute to the induction of LIRE is a matter of ongoing controversy [10] , [11] , [22] , [23] , [24] . We thus examined whether the role of NADPH oxidase in circulating and resident leukocytes was different from that of NADPH oxidase in endothelial cells. To this end, we created chimeric mice by transplanting Nox2 y/− bone marrow cells into lethally irradiated WT mice ( Nox2 y/− to WT chimera) and vice versa (WT to Nox2 y/− chimera). Isolated lungs from Nox2 y/− to WT chimeras showed an increase in lung weight ( Supplementary Fig. S1c ) and Kfc values ( Supplementary Fig. S1d ) following ischaemia–reperfusion, similar to lungs from non-chimeric WT mice and control WT mice transplanted with WT bone marrow (WT to WT chimera). However, WT to Nox2 y / − chimeric mice did not develop increased vascular permeability after ischaemia–reperfusion ( Supplementary Fig. S1c,d ). Moreover, Nox2-deficency exclusively in the myeloid lineage resulted in lung weight gain and increased Kfc values similar to WT conditions, whereas endothelial cell-specific Nox2 inactivation protected from LIRE ( Fig. 1e–h ). Therefore, it is the endothelial Nox2 function that is most likely responsible for the induction of LIRE. Consistently, bronchoalveolar lavage cells from Nox2 y/− and myeloid Nox2-deficient mice did not release superoxide upon NADPH oxidase stimulation, whereas those from WT mice did ( Supplementary Fig. S2 ). To elucidate the role of TRPC6 in LIRE, we analysed TRPC6 − / − mice in a way similar to that described for Nox2 y / − mice. Lungs isolated from TRPC6 − / − mice displayed no significant changes in weight gain ( Fig. 2a ) and Kfc values ( Fig. 2b ) following ischaemia–reperfusion. 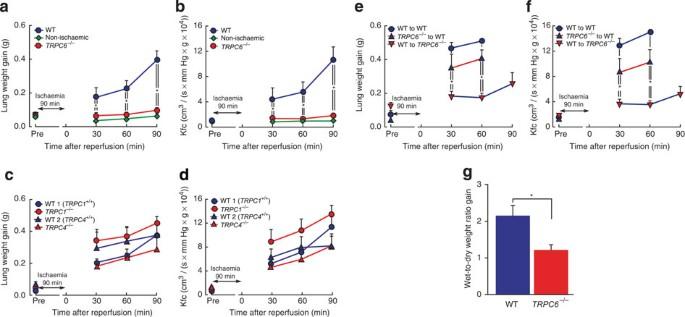Figure 2: Analysis of LIRE in WT andTRPC-deficient (TRPC1−/−,TRPC4−/−andTRPC6−/−) lungs. (a,b) Post-ischaemic vascular leakage in isolated lungs of WT andTRPC6−/−mice, (c,d) TRPC1- and TRPC4-deficient animals, and (e,f) chimeric mice. (g) Analysis of ischaemia–reperfusion-induced pulmonary oedema formation in living mice. (a,c,e) Lung weight gain was calculated as the weight difference before and after each hydrostatic challenge manoeuvre. (b,d,f). The lung Kfc was determined before ischaemia and at 30-min intervals after re-establishing perfusion. (e,f) Post-ischaemic vascular leakage in isolated lungs of chimeric mice, in which bone marrow cells of WT orTRPC6−/−mice were transplanted to irradiated WT mice, or bone marrow cells ofTRPC6−/−to irradiated WT mice. If 90-min values are not displayed, experiments had to be terminated before, because of excessive oedema formation. (g) Pulmonary oedema formation in living mice was analysed by quantitative assessment of wet-to-dry weight ratios of ischaemia-exposed lungs normalized to sham-operated mice. (a–g)n=4–7. Data were statistically analysed by Student'st-test with Welsh's correction for comparison of two groups and one-way analysis of variance with the Student–Newman–Keuls test for multiple comparisons. All data are presented as mean±s.e.m.; *P<0.05. Figure 2: Analysis of LIRE in WT and TRPC -deficient ( TRPC1 − / − , TRPC4 − / − and TRPC6 − / − ) lungs. ( a , b ) Post-ischaemic vascular leakage in isolated lungs of WT and TRPC6 − / − mice, ( c , d ) TRPC1- and TRPC4-deficient animals, and ( e , f ) chimeric mice. ( g ) Analysis of ischaemia–reperfusion-induced pulmonary oedema formation in living mice. ( a , c , e ) Lung weight gain was calculated as the weight difference before and after each hydrostatic challenge manoeuvre. ( b , d , f ). The lung Kfc was determined before ischaemia and at 30-min intervals after re-establishing perfusion. ( e , f ) Post-ischaemic vascular leakage in isolated lungs of chimeric mice, in which bone marrow cells of WT or TRPC6 − / − mice were transplanted to irradiated WT mice, or bone marrow cells of TRPC6 − / − to irradiated WT mice. If 90-min values are not displayed, experiments had to be terminated before, because of excessive oedema formation. ( g ) Pulmonary oedema formation in living mice was analysed by quantitative assessment of wet-to-dry weight ratios of ischaemia-exposed lungs normalized to sham-operated mice. ( a – g ) n =4–7. Data were statistically analysed by Student's t -test with Welsh's correction for comparison of two groups and one-way analysis of variance with the Student–Newman–Keuls test for multiple comparisons. All data are presented as mean±s.e.m. ; * P <0.05. Full size image The specific contribution of TRPC6 to pulmonary oedema is underlined by the fact that lungs from TRPC1- [25] and TRPC4-deficient mice [26] were not protected from increased vascular permeability caused by ischaemia–reperfusion ( Fig. 2c,d ). To differentiate between the role of TRPC6 in circulating and resident leukocytes versus that in endothelial cells, TRPC6 − / − bone marrow cells were transplanted into lethally irradiated WT mice ( TRPC6 − / − to WT chimera) and vice versa (WT to TRPC6 − / − chimera; Supplementary Methods ). Isolated lungs from TRPC6 − / − to WT chimeric mice responded to ischaemia–reperfusion with a lung weight gain ( Fig. 2e ) and increased Kfc values ( Fig. 2f ), similarly to lungs from non-chimeric WT mice and WT to WT chimeras. By contrast, WT to TRPC6 − / − chimeric mice did not develop increased vascular permeability after hydrostatic challenge ( Fig. 2e,f ), suggesting that TRPC6 function in non-bone marrow-derived cells—and thus likely in endothelial cells—is important for the development of LIRE. Moreover, TRPC6 − / − mice were also protected from lung oedema formation caused by ischaemia–reperfusion in vivo ( Fig. 2g ). For details and variations of the ischaemia–reperfusion protocol, see Materials and Methods and Supplementary Figure S3 . The extent of protection from LIRE was very similar between Nox2 y / − and TRPC6 − / − mice. On the basis of recent findings that TRPC6 represents a target for ROS derived from NADPH oxidases [17] , [18] , [19] , we reasoned that Nox2 and TRPC6 proteins might be components of the same signal transduction pathway leading to lung oedema. Nox2 produces superoxide raising [(Ca 2 + ) i ] via TRPC6 To investigate the role of Nox2 and TRPC6 at the cellular level, we isolated primary murine lung endothelial cells (MLEC) from WT, Nox2 y/− and TRPC6 −/− mice. MLEC were identified by staining with antibodies directed against von Willebrand factor and platelet endothelial cell adhesion molecule-1 ( Fig. 3a ). In immunoblots using a TRPC6-specific antiserum, TRPC6 protein was detected in lysates of WT endothelial cells, but not in TRPC6 − / − endothelial cells ( Fig. 3b ). As TRPC6 deficiency might be compensated for by upregulation of closely related members of the TRPC family [27] , we assessed the expression of TRPC subtypes in primary MLEC. Quantitative reverse-transcription PCR analysis revealed predominant expression of TRPC1, TRPC4 and TRPC6 mRNA in MLEC from WT mice ( Supplementary Methods ). A compensatory upregulation of other TRPC subtypes in TRPC6 − / − MLEC was not observed ( Supplementary Figure S4a ). Moreover, hypoxia or application of H 2 O 2 did not induce any changes in the TRPC-expression pattern in WT endothelial cells ( Supplementary Fig. S4b ), nor did H 2 O 2 (100 μM) activate TRPC6 directly in endothelial cells. 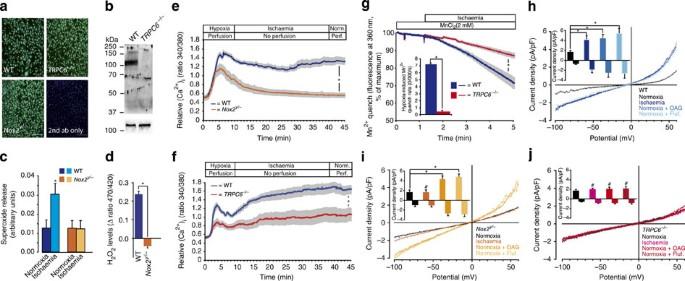Figure 3: Characterization of WT, Nox2-deficient (Nox2y/−) and TRPC6-deficient (TRPC6−/−) primary MLEC. (a) Identification of MLEC (WT, wild-type; TRPC6−/−, TRPC6-deficient; Nox2−/−, Nox2-deficient; 2nd ab only, only second antibody applied) cultured for 7 days. Cells were stained with antibodies against platelet endothelial cell adhesion molecule-1 (PECAM-1 ab). Scale bars correspond to 200 μm. (b) Immunoblotting of cell lysates extracted from WT andTRPC6−/−MLEC, and detection of TRPC6 protein using a TRPC6-specific antiserum. (Lower part) An imunoblot detecting vinculin serves as a loading control. (c) Extracellular superoxide release after 30 min of ischaemia or normoxia in MLEC. (d) Differences in intracellular H2O2levels in MLEC induced by ischaemia–reperfusion and detected by the HyPer sensor. (e) Increase in the [Ca2+]iupon ischaemia–reperfusion (Norm., Perf.). (f) Cation influx in MLEC from WT andTRPC6−/−mice. Increase in the [Ca2+]iupon ischaemia–reperfusion (Norm., Perf.). (g) Ischaemia-induced Mn2+influx inTRPC6−/−and WT MLEC. (Inset) Summary of Mn2+influx experiments. (h–j) Representative current density–voltage relationships during normoxia and hypoxia, as well as during application of a membrane-permeable analogue of diacylglycerol (OAG, 100 μM) and of flufenamic acid, an activator of TRPC6 (Fluf., 100 μM), under normoxic conditions are displayed. (Insets) Summaries of current densities–voltage relationships at holding potentials of ±60 mV. (c)n=6–7 independent experiments. (d–f)n=56–172 cells. (g)n=9–10 cells. (h–j)n=6–10 cells. All statistical data were assessed using Student'st-test with Welsh's correction and are presented as mean±s.e.m.; *P<0.05. (h–j)n=6–10 cells. The data are presented as mean±s.e.m. Paired Student'st-test was used for comparison with normoxia. Unpaired Student'st-test was used for comparison with WT MLEC;*,#P<0.05. Figure 3: Characterization of WT, Nox2-deficient (Nox2 y/ − ) and TRPC6-deficient (TRPC6 − / − ) primary MLEC. ( a ) Identification of MLEC (WT, wild-type; TRPC6 − / − , TRPC6-deficient; Nox2 − / − , Nox2-deficient; 2nd ab only, only second antibody applied) cultured for 7 days. Cells were stained with antibodies against platelet endothelial cell adhesion molecule-1 (PECAM-1 ab). Scale bars correspond to 200 μm. ( b ) Immunoblotting of cell lysates extracted from WT and TRPC6 −/− MLEC, and detection of TRPC6 protein using a TRPC6-specific antiserum. (Lower part) An imunoblot detecting vinculin serves as a loading control. ( c ) Extracellular superoxide release after 30 min of ischaemia or normoxia in MLEC. ( d ) Differences in intracellular H 2 O 2 levels in MLEC induced by ischaemia–reperfusion and detected by the HyPer sensor. ( e ) Increase in the [Ca 2+ ] i upon ischaemia–reperfusion (Norm., Perf.). ( f ) Cation influx in MLEC from WT and TRPC6 − / − mice. Increase in the [Ca 2+ ] i upon ischaemia–reperfusion (Norm., Perf.). ( g ) Ischaemia-induced Mn 2+ influx in TRPC6 − / − and WT MLEC. (Inset) Summary of Mn 2+ influx experiments. ( h – j ) Representative current density–voltage relationships during normoxia and hypoxia, as well as during application of a membrane-permeable analogue of diacylglycerol (OAG, 100 μM) and of flufenamic acid, an activator of TRPC6 (Fluf., 100 μM), under normoxic conditions are displayed. (Insets) Summaries of current densities–voltage relationships at holding potentials of ±60 mV. ( c ) n =6–7 independent experiments. ( d – f ) n =56–172 cells. ( g ) n= 9–10 cells. ( h – j ) n =6–10 cells. All statistical data were assessed using Student's t -test with Welsh's correction and are presented as mean±s.e.m. ; * P <0.05. ( h – j ) n =6–10 cells. The data are presented as mean±s.e.m. Paired Student's t -test was used for comparison with normoxia. Unpaired Student's t -test was used for comparison with WT MLEC; *,# P <0.05. Full size image In line with our findings in intact lungs, WT cells reacted to ischaemic conditions with superoxide release into the extracellular medium, whereas Nox2 y/− MLEC were unresponsive ( Fig. 3c ) when compared with normoxic conditions as monitored by electron spin resonance (ESR) spectroscopy applying an extracellular spin probe. Using the H 2 O 2 -specific HyPer detection method, WT cells displayed a rise of intracellular H 2 O 2 levels after ischaemia–reperfusion. This increase was completely abolished in Nox2 y/− MLEC ( Fig. 3d ). In line with the assumption of extracellularly released superoxide being converted to H 2 O 2 , diffusing into MLEC to increase intracellular H 2 O 2 levels in ischaemia, extracellular catalase significantly reduced, but extracellular superoxide dismutase increased intracellular H 2 O 2 levels ( Supplementary Fig. S5a ). This finding was further substantiated by employing amplex red as a fluorescence probe specific for extracellular H 2 O 2 ( Supplementary Fig. S5d ). Moreover, our data show that ROS levels were already rising during ischaemia, but do not further increase during reperfusion ( Supplementary Fig. S5a–c ). In addition, after ischaemia–reperfusion, [Ca 2+ ] i was significantly decreased in Nox2 y/− cells compared with WT cells ( Fig. 3e ), prompting us to investigate Ca 2+ entry pathways in MLEC ( Supplementary Methods ). The increase in [Ca 2+ ] i elicited by ischaemic incubation of WT MLEC was significantly decreased in MLEC from TRPC6 − / − mice ( Fig. 3f ). To differentiate between Ca 2+ influx and release of Ca 2+ from internal stores, we monitored TRPC6 activity in MLEC by analysing ischaemia-induced Mn 2+ influx. Ischaemia initiated a marked influx of cations from the extracellular space in WT, but not in TRPC6 − / − MLEC ( Fig. 3g and inset). As store-operated Ca 2+ channels and capacitative calcium entry through TRPC4 have been suggested to contribute to the regulation of [Ca 2+ ] i in endothelial cells [4] , [5] , we investigated the role of internal Ca 2+ stores in the ischaemia-induced increase in [Ca 2+ ] i . In contrast to previous reports [4] , [5] , we found that ischaemia-induced elevation of [Ca 2+ ] i does not depend on Ca 2+ release from internal stores, because ischaemia-induced increases in [Ca 2+ ] i were not detectable in the absence of extracellular Ca 2+ ( Supplementary Fig. S6a ). However, both WT and TRPC6 − / − cells responded to thapsigargin by a comparable Ca 2+ release from intracellular stores ( Supplementary Fig. S6b ). Endothelial cells are generally viewed as being electrically non-excitable. In keeping with this notion, addition of nicardipine (10 μM) to isolated lungs failed to prevent LIRE in WT lungs, whereas SKF-96365 (50 μM), an inhibitor of receptor-mediated Ca 2+ entry, significantly reduced vascular permeability ( Supplementary Fig. S7 ). To assess ischaemia-induced membrane currents through TRPC channels directly, we measured cationic currents in MLEC ( Supplementary Methods ). Ischaemia increased both inward and outward currents in MLEC from WT mice ( Fig. 3h ), but not in MLEC from Nox2 y /− and TRPC6 −/− mice ( Fig. 3i,j ). Under normoxic conditions, exposure to oleoylacetylglycerol (OAG), a membrane-permeable analogue of the TRPC3/6/7 channel activator DAG, as well as the TRPC6 activator flufenamic acid, resulted in a significant increase in current densities in MLEC from WT and Nox2 y/− mice ( Fig. 3i,j ), but not in those from TRPC6 −/− mice ( Fig. 3j ). TRPC6 controls endothelial cell permeability Changes in endothelial barrier function were determined by analysing cellular resistance of WT and TRPC6 −/− endothelial cells under flow conditions. Cellular resistance was profoundly decreased in response to ischaemia in WT MLEC, whereas TRPC6 −/− and Nox2 y/− MLEC were significantly less affected ( Fig. 4a ). The TRPC6 activator OAG was able to increase endothelial permeability in WT and Nox2 y/− MLEC, but not in TRPC6 −/− cells ( Fig. 4b ). Moreover, MLEC from TRPC6 −/− mice expressing a recombinant TRPC6 fused to the enhanced green fluorescent protein (eGFP) reacted to ischaemia with a significantly pronounced decrease in cell monolayer resistance, compared with cells transfected with eGFP cDNA alone, emphasizing an essential role of TRPC6 for endothelial cell shape change ( Fig. 4c ). 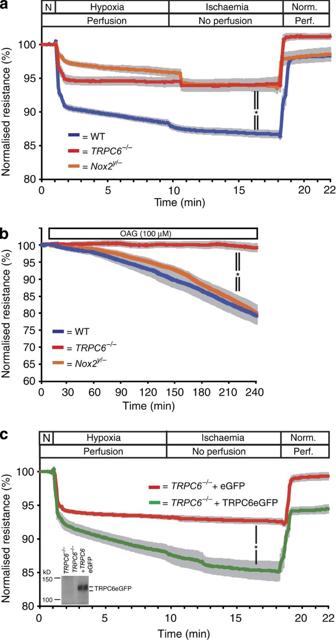Figure 4: Endothelial cell function in MLEC isolated from WT, Nox2- (Nox2y/−) and TRPC6-deficient (TRPC6−/−) mice. (a) Analysis of ischaemia-induced changes in cell resistance in WT,Nox2y/−andTRPC6−/−endothelial cells using ECIS analysis under flow conditions. (b) Application of OAG to WT,Nox2y/−and TRPC6−/−cells in an array chamber. (c)TRPC6−/−cells electroporated with plasmids coding for the eGFP or TRPC6 fused to eGFP (TRPC6eGFP) were analysed by an electrical impedance sensor (ECIS). (Inset) Immunoblot ofTRPC6−/−MLEC and TRPC6eGFP-transfectedTRPC6−/−MLEC. (a–c)n=4 independent experiments. N. Norm., normoxia; Perf., perfusion. All statistical data were assessed using Student'st-test with Welsh's correction and are presented as mean±s.e.m.; *P<0.05. Figure 4: Endothelial cell function in MLEC isolated from WT, Nox2- (Nox2 y/− ) and TRPC6-deficient (TRPC6 − / − ) mice. ( a ) Analysis of ischaemia-induced changes in cell resistance in WT, Nox2 y/− and TRPC6 −/− endothelial cells using ECIS analysis under flow conditions. ( b ) Application of OAG to WT, Nox2 y /− and TRPC6 −/− cells in an array chamber. ( c ) TRPC6 − / − cells electroporated with plasmids coding for the eGFP or TRPC6 fused to eGFP (TRPC6eGFP) were analysed by an electrical impedance sensor (ECIS). (Inset) Immunoblot of TRPC6 −/− MLEC and TRPC6eGFP-transfected TRPC6 −/− MLEC. ( a – c ) n =4 independent experiments. N. Norm., normoxia; Perf., perfusion. All statistical data were assessed using Student's t -test with Welsh's correction and are presented as mean±s.e.m. ; * P <0.05. Full size image Involvement of PLCγ phosphorylation in LIRE To identify further proteins and signalling steps involved in the transduction cascade from the production of ROS by Nox2 to the activation of TRPC6 channels, we examined the effect of a PLC inhibitor on LIRE in isolated lungs. Although the active PLC inhibitor (U73122) completely abolished LIRE, an inactive analogue (U73343) did not suppress LIRE ( Fig. 5a,b ). In vivo , anaesthetized WT mice exposed to the solvent dimethyl sulfoxide developed severe lung oedema following ischaemia–reperfusion; however, U73122-treated WT mice were protected ( Fig. 5c ). In additional experiments, we excluded any inhibitory effects of U73122 on TRPC6 activity. 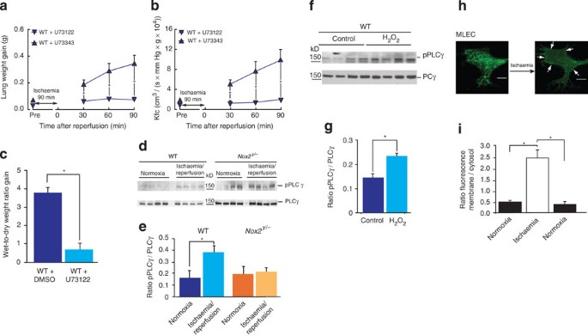Figure 5: Activation of C-type phospholipase (PLC) and accumulation of DAG during ischaemia–reperfusion in isolated lungs and MLEC. (aandb) Post-ischaemic vascular leakage in isolated lungs of WT mice undergoing ischaemia–reperfusion with application of the PLC inhibitor U73122 and its non-functional analogue U73343. (a) WT lung weight gain. (b) Lung Kfc of WT lungs. (c) Pulmonary oedema formation in living mice ±U73122 normalized to sham-operated mice. (d) Immunoblot of protein lysates of normoxic and ischaemic lungs from WT (WT) and Nox2-deficient (Nox2y/−) mice with a phosphospecific PLCγ antibody (pPLCγ) and a PLCγ antibody (e) Quantitative analysis of PLCγ phosphorylation. (f) Immunoblot of protein lysates of MLEC±H2O2(100 μM; for 5 min) incubated with a pPLCγ and a PLCγ antibody. (g) Quantitative analysis of PLCγ phosphorylation in control MLEC and MLEC treated with H2O2. (h) Fluorescence images of MLEC expressing a fluorescent DAG sensor. Scale bars correspond to 10 μm and arrows are indicating plasma membrane staining. (i) Summarized data for the ratios of plasma membrane versus cytosolic fluorescence intensities of WT MLEC. (a–c)n=5. (i)n=5 cells. All statistical data were assessed using Student'st-test with Welsh's correction and are presented as mean±s.e.m.; *P<0.05. Figure 5: Activation of C-type phospholipase (PLC) and accumulation of DAG during ischaemia–reperfusion in isolated lungs and MLEC. ( a and b ) Post-ischaemic vascular leakage in isolated lungs of WT mice undergoing ischaemia–reperfusion with application of the PLC inhibitor U73122 and its non-functional analogue U73343. ( a ) WT lung weight gain. ( b ) Lung Kfc of WT lungs. ( c ) Pulmonary oedema formation in living mice ±U73122 normalized to sham-operated mice. ( d ) Immunoblot of protein lysates of normoxic and ischaemic lungs from WT (WT) and Nox2-deficient ( Nox2 y/− ) mice with a phosphospecific PLCγ antibody (pPLCγ) and a PLCγ antibody ( e ) Quantitative analysis of PLCγ phosphorylation. ( f ) Immunoblot of protein lysates of MLEC±H 2 O 2 (100 μM; for 5 min) incubated with a pPLCγ and a PLCγ antibody. ( g ) Quantitative analysis of PLCγ phosphorylation in control MLEC and MLEC treated with H 2 O 2 . ( h ) Fluorescence images of MLEC expressing a fluorescent DAG sensor. Scale bars correspond to 10 μm and arrows are indicating plasma membrane staining. ( i ) Summarized data for the ratios of plasma membrane versus cytosolic fluorescence intensities of WT MLEC. ( a – c ) n =5. ( i ) n =5 cells. All statistical data were assessed using Student's t -test with Welsh's correction and are presented as mean±s.e.m. ; * P <0.05. Full size image As phosphorylation and subsequent activation of PLCγ by H 2 O 2 has been shown in renal artery vascular smooth muscle cells [28] , we investigated whether this also occurs in lungs using a phosphorylation-specific PLCγ antibody. Only moderate levels of phosphorylated PLCγ were detectable during normoxia, but ischaemia–reperfusion induced a significant increase in phosphorylated PLCγ in WT, but not in Nox2 -deficient lungs ( Fig. 5d,e ). Moreover, H 2 O 2 was able to induce PLCγ phosphorylation in MLEC ( Fig. 5f,g ). Like all other PLC isozymes, PLCγ cleaves phosphatidylinositol-4,5-bisphosphate into inositol-1,4,5-trisphosphate and DAG. Therefore, we investigated whether ischaemia would induce DAG accumulation at the plasma membrane of endothelial cells, necessary to activate TRPC6. We took advantage of a fluorescent DAG-sensor, consisting of the DAG-binding C1 domain of protein kinase Cδ [29] fused to eGFP, to monitor changes in the local distribution of cellular DAG contents in response to ischaemia. In WT MLEC, the DAG sensor was localized in the cytosol under normoxic conditions, but under ischaemic conditions, DAG-dependent fluorescence redistributed to the plasma membrane ( Fig. 5h,i ). This effect was fully reversible after normoxic perfusion ( Fig. 5i ). DAG kinase activity reduces ischaemia-reperfusion-induced TRPC6 activation DAG is an important second messenger in the cell and is rapidly degraded by cellular enzymes. In particular, DAG kinases metabolize DAG to phosphatidic acid [30] , representing the main route to inactivate DAG. To analyse the role of DAG kinases in LIRE, we used R59949, a potent enzyme inhibitor. Application of R59949 resulted in a rise of [Ca 2+ ] i in WT MLEC, whereas TRPC6 − / − MLEC were completely unresponsive ( Fig. 6a ). As these data point to a role of DAG kinases in the regulation of TRPC6 activity, we analysed the expression pattern of DAG kinases in endothelial cells. Among the DAG kinases tested, the α and η isozymes were prominently expressed in endothelial cells ( Fig. 6b ). Using an in vitro assay ( Supplementary Methods ) in which the DAG kinase isoforms α, β, γ and η are expressed heterologously in HEK293 cells, we analysed their sensitivity to H 2 O 2 . Although metabolism of DAG by the α, β and γ isoforms was unchanged after application of H 2 O 2 , the enzymatic activity of both η isoforms was markedly inhibited ( Fig. 6c ). Therefore, we overexpressed exogenous DAG kinase η 1 and η 2 isoforms fused to eGFP in WT MLEC and assessed Ca 2+ influx following ischaemia–reperfusion in these cells in comparison with cells transfected with the eGFP cDNA alone. As expected, expression of DAG kinase η 1+2 was able to suppress [Ca 2+ ] i increases in endothelial cells ( Fig. 6d ). 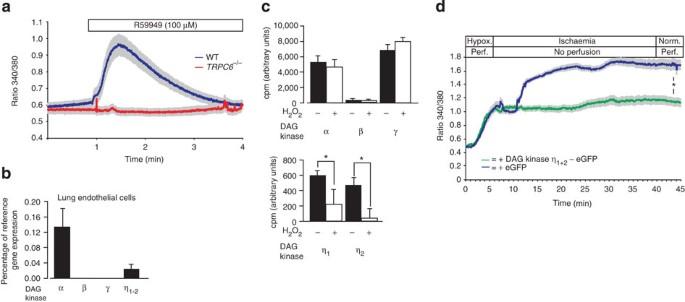Figure 6: Influence of DAG kinase activity on ischaemia-induced increases in [Ca2+]i. (a) Effects of the DAG kinase inhibitor II (R59949) on the [Ca2+]iin WT versusTRPC6-deficient (TRPC6−/−) MLEC. (b) Quantification of mRNAs encoding DAG kinases to β-actin (as reference gene) with the aid of a light cycler. (c)In vitroassay for DAG kinase α, β, γ and η activity±pre-incubation with H2O2(100 μM). (d) Cation influx in MLEC from WT cells electroporated with DAG kinase η1and η2fused to the eGFP (+DAG kinase η1+2-eGFP) and eGFP alone (+eGFP). N. Norm., normoxia; Perf., perfusion. (a)n=42–61 cells (b) MLEC fromn=5 mice. (c)n=3 independent experiments. (d)n=76–104 cells. All statistical data were assessed using Student'st-test with Welsh's correction and are presented as mean±s.e.m.; *P<0.05. Figure 6: Influence of DAG kinase activity on ischaemia-induced increases in [Ca 2+ ] i . ( a ) Effects of the DAG kinase inhibitor II (R59949) on the [Ca 2+ ] i in WT versus TRPC6 -deficient ( TRPC6 − / − ) MLEC. ( b ) Quantification of mRNAs encoding DAG kinases to β-actin (as reference gene) with the aid of a light cycler. ( c ) In vitro assay for DAG kinase α, β, γ and η activity±pre-incubation with H 2 O 2 (100 μM). ( d ) Cation influx in MLEC from WT cells electroporated with DAG kinase η 1 and η 2 fused to the eGFP (+DAG kinase η 1+2 -eGFP) and eGFP alone (+eGFP). N. Norm., normoxia; Perf., perfusion. ( a ) n =42–61 cells ( b ) MLEC from n =5 mice. ( c ) n =3 independent experiments. ( d ) n =76–104 cells. All statistical data were assessed using Student's t -test with Welsh's correction and are presented as mean±s.e.m. ; * P <0.05. Full size image To further substantiate our hypothesis that both DAG accumulation by PLCγ and DAG kinase inhibition are essential for TRPC6 activation in the early stages of LIRE, we examined isolated WT lungs after ischaemia–reperfusion or normoxia in the presence of OAG and/or DAG-kinase inhibitor. OAG enhanced ischaemia–reperfusion-induced vascular permeability significantly in isolated WT lungs and induced lung oedema in Nox2 y/− mice during ischaemia–reperfusion, compared with lungs treated with the solvent dimethyl sulfoxide ( Fig. 7a,b ). Furthermore, non-ischaemic lungs developed oedema comparable to LIRE lungs when both OAG and DAG-kinase inhibitor were applied ( Fig. 7a,b ). 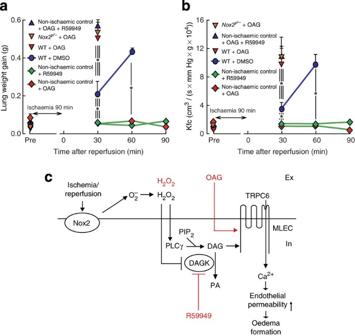Figure 7: Influence of pharmacological tools on lung ischaemia–reperfusion-induced oedema (LIRE). (a,b) Post-ischaemic vascular leakage in isolated WT andNox2y/−lungs undergoing ischaemia–reperfusion or normoxia±OAG and/or DAG-kinase inhibitor R59949. Lungs were exposed to ischaemia or normoxia for 90 min. (a) Lung weight gain. (b) Lung Kfc. If 60- or 90-min values are not displayed experiments had to be terminated before due to excessive oedema formation. (c) Proposed signal transduction cascade in LIRE. Pharmacological interventions are indicated in red. DAG, diacylglycerol; Ex, extracellular; In, intracellular; OAG, Oleoylacetylglycerol; PA, phosphatidic acid; PIP2, phosphatidylinositol 4,5-bisphosphate. (a,b)n=5 lungs each. Data were statistically analysed by analysis of variance with the Student–Newman–Keuls test. All data are presented as mean±s.e.m.; *P<0.05. Figure 7: Influence of pharmacological tools on lung ischaemia–reperfusion-induced oedema (LIRE). ( a , b ) Post-ischaemic vascular leakage in isolated WT and Nox 2 y/− lungs undergoing ischaemia–reperfusion or normoxia±OAG and/or DAG-kinase inhibitor R59949. Lungs were exposed to ischaemia or normoxia for 90 min. ( a ) Lung weight gain. ( b ) Lung Kfc. If 60- or 90-min values are not displayed experiments had to be terminated before due to excessive oedema formation. ( c ) Proposed signal transduction cascade in LIRE. Pharmacological interventions are indicated in red. DAG, diacylglycerol; Ex, extracellular; In, intracellular; OAG, Oleoylacetylglycerol; PA, phosphatidic acid; PIP 2 , phosphatidylinositol 4,5-bisphosphate. ( a , b ) n =5 lungs each. Data were statistically analysed by analysis of variance with the Student–Newman–Keuls test. All data are presented as mean±s.e.m. ; * P <0.05. Full size image Impaired endothelial barrier function with subsequent oedema formation and organ failure is the characteristic feature in early stages of LIRE. However, the molecular steps involved in the loss of endothelial integrity and subsequent oedema formation are still poorly understood. We report evidence to support a mechanistic model of LIRE in mice involving a sequence of events starting with increased endothelial ROS production by activated endothelial Nox2, leading to PLCγ activation, DAG kinase inhibition and subsequent DAG-mediated TRPC6 activation. To differentiate between the role of Nox2 in leukocytic versus endothelial cells, Nox2 y / − bone marrow cells were transplanted into lethally irradiated WT mice and vice versa. Next, we investigated mice deficient of Nox2 in cells of the myeloid lineage or specifically in endothelial cells. These experiments supported the notion that endothelial, but not leukocytic Nox2, function protects from LIRE. Corresponding results were obtained with chimeric TRPC6 −/− mice. The results from the ex-vivo lung experiments were corroborated in an in-vivo mouse lung ischaemia–reperfusion model. These findings are in contrast to findings that depletion of alveolar macrophages protects against LIRE [10] , [31] . However, depletion of macrophages by clodronate liposomes or gadolinium chloride can have effects beyond macrophage depletion, like inhibition of ion channels and an increase in the lung-surfactant pool, which can explain protection from LIRE besides the effect on macrophages [32] , [33] , [34] , [35] , [36] , [37] . Although we show a complete protection from LIRE by deletion of endothelial Nox2, Yang et al . [24] recently showed partial protection from LIRE by deletion of p47 phox in bone marrow cells. This partial effect on LIRE may be explained by the fact that lungs were exposed to a much shorter ischaemic period, so that injury particularly in early reperfusion was much milder than in our experiments. Along these lines, it can be suggested that endothelial Nox2 triggers the initial event of LIRE and that bone marrow-derived NADPH oxidases have an additional role in the later stages of LIRE when secondary neutrophil invasion can occur after endothelial injury. Moreover, compensatory effects of p47 phox deficiency even after bone marrow transplantation cannot be excluded. In contrast, such effects are most unlikely in our inducible endothelial cell-specific Nox2-knockout mice. To decipher the underlying signalling cascade of LIRE, we next demonstrated a lack of intravascular superoxide release in Nox2 y / − mice during ischaemia–reperfusion. Focusing on primary endothelial cells from Nox2 y/− mice and the corresponding WT strain, we confirmed extracellular superoxide production during ischaemia–reperfusion. Possibly, activation of Nox2 during ischaemia occurs via Rac1 activation or mechanotransduction and membrane depolarization [38] , [39] , [40] . Measurement of intra- and extracellular H 2 O 2 levels upon application of extracellular superoxide dismutase or catalase, suggested that extracellular superoxide is converted to H 2 O 2 and induces ischaemia–reperfusion-induced increase of vascular permeability upon diffusion into MLEC. Moreover, our data indicate that H 2 O 2 already starts to increase during ischaemia, consistent with a similar kinetics of the [Ca 2+ ] i rise found in MLEC. In TRPC6-deficient endothelial cells, the rise in [Ca 2+ ] i was attenuated when compared with WT cells. Contrary to previous reports (reviewed in Mehta and Malik [41] ), emptying of internal calcium stores was not responsible for the rise in ischaemia–reperfusion-induced [Ca 2+ ] i as shown by our experiments under conditions of extracellular Ca 2+ deprivation. In this context, it is important to mention that members of the TRPC family can act as receptor-operated or store-operated channels and have been identified in endothelial cells by several research groups [41] , [42] , [43] . The exclusive role of TRPC6 channels in LIRE was further confirmed by the fact that deletion of other TRPC channels, TRPC1 and TRPC4, which are also prominently expressed in lung endothelial cells, do not protect from LIRE in the intact organ. To address the issue as to how Nox2-mediated ROS generation activates TRPC6 channels during LIRE, we subsequently focused on DAG. It has previously been demonstrated that TRPC6 can be activated by DAG and that the DAG-generating PLC isoenzyme PLCγ can be stimulated by H 2 O 2 [28] . We found that activated phospho-PLCγ was increased in lungs exposed to ischaemia–reperfusion, as well as in MLEC, after exposure to H 2 O 2 . PLCγ phosphorylation in ischaemia–reperfusion was dependent on Nox2 function, as it was not found in Nox2 y/− lungs. Moreover, application of ischaemia to endothelial cells resulted in DAG accumulation, which is at least partially caused by the inhibition of DAG kinase η isoforms, degrading DAG to phosphatidic acid [44] . OAG administration and DAG kinase inhibition in intact lungs mimicked DAG accumulation and consequently LIRE in normoxic lungs. Furthermore, OAG reversed the protection against ischaemia–reperfusion-induced increase of vascular permeability in Nox2 y / − mice. In conclusion, Nox2 and TRPC6 have a hitherto unappreciated, indispensable role in the development of LIRE in mice. Deciphering the signalling cascade from Nox2 activation to ROS-mediated, DAG-dependent TRPC6 activation and subsequent increases in lung endothelial permeability and oedema (summarized in Fig. 7c ) provides new insight into the pathophysiology of the early stages of LIRE. If future experiments in human lungs indicate that our findings are transferable to the human situation, this may offer new promising strategies to suppress the progression of LIRE in the clinical setting. Animals All animal experiments were approved by the governmental authorities (Regierungspräsidium Giessen). As genes for Nox1 and Nox2 are located on the X chromosome, male mice carrying a mutated allele on their single X chromosomes were used and labelled as Nox1 y/− and Nox2 y/− mice throughout the manuscript. TRPC6 − / − , Nox1 y/− and Nox4 −/− mice were generated as previously described [27] , [45] , [46] . C57Bl/6 and Nox2 y/− mice were purchased from Jackson Laboratories [21] . Mice deficient for Nox2 either in cells of the myeloid lineage or tamoxifen-inducible in endothelial cells were generated by crossing C57BL/6-TG-Nox2 Flox/Flox with the appropriate Cre-deleter mice. Generation of mice deficient for Nox2 Mice deficient for Nox2 either in cells of the myeloid lineage or tamoxifen-inducible in endothelial cells were generated by crossing C57BL/6-TG-Nox2- Flox/Flox C57BL/6-TG-Lysm-Cre+/0 and C57BL/6-TG-ERT2-Tie2-Cre+/0, respectively, as provided by the co-authors [47] . Offsprings were crossed and bred homozygous for the Flox allele and by mating 0/+×0/0 of the Cre-line in the Flox-background hemizygous or null for the Cre construct. To induce endothelial-specific deletion of Nox2, mice receive injections of tamoxifen (40 mg kg −1 , 100 μl intraperitoneally of a solution of 1 mg ml −1 tamoxifen dissolved in 90% corn oil, 10% ethanol) on three consecutive days and experiments were performed 7 days after the last tamoxifen injection. Analysis of ischaemia–reperfusion-induced oedema in living mice The Nox2 y /− , TRPC6 −/− or corresponding WT mice were anaesthetized by intraperitoneal injection of ketamine (100 mg kg −1 ) and xylazine (8 mg kg −1 ). Mice were placed in a heating chamber to maintain body temperature (37 °C) during the entire experiment. Endotracheal intubation with a 21-gauge atraumatic cannula was performed by tracheotomy, and mechanical ventilation was initiated (130 breaths per min, 225 μl stroke volume, and a positive-end expiratory pressure of 2 cm H 2 O) with an inspiratory oxygen fraction of 50%, using a mouse ventilator MiniVent type 845 (Hugo Sachs Elektronik, March-Hugstetten, Germany). After a left anterolateral thoracotomy through the third left intercostal space, all animals were given 500 IU kg −1 heparin. Five minutes after heparin administration, the pulmonary hilum of the left lung, including the bronchus, pulmonary artery and pulmonary vein, was occluded for 90 min using a non-crushing microsurgical clamp to cause pulmonary ischaemia of the left lung in an inflated state. Upon removal of the clamp, the left lung was reperfused and reventilated for 90 min. The PLC inhibitor U-73122 (2.5 mg kg −1 ) or vehicle were administered to WT mice via tail vein 10 min before starting ischaemia. In time-matched sham-operated animals serving as controls, thoracotomy was performed without occlusion of the hilum. In this group, U-73122 or vehicle were administered into WT mice via the tail vein at a time point corresponding to that in ischaemia–reperfusion groups. At the end of the reperfusion period, animals were killed, and left lungs were excised for assessment of tissue water content. As a measure of pulmonary oedema formation, wet-to-dry lung weight ratios were determined for left lungs. For this purpose, total lung weight was measured before (wet weight) and after a 48-h drying process (dry weight) and values were normalized to sham-operated controls. Isolation and culture of murine endothelial cells MLEC were isolated from the lungs of five mice (WT and TRPC6 − / − ). After explantation of the lungs, tissue slices of 1 mm were prepared in a cell culture hood and washed in Hanks' balanced salt solution (HBSS, containing 140 mM NaCl, 5 mM KCl, 1 mM MgCl 2 , 2 mM CaCl 2 , 5 mM glucose in 10 mM 4-(2-hydroxyethyl)-1-piperazineethanesulfonic acid (HEPES) buffer (pH 7.4)) to remove remaining blood. Minced tissues were transferred to a sterile 50-ml tube containing 20 ml HBSS without Ca 2+ and Mg 2+ and dispase (1 U ml −1 ), and digested for 60 min at 37 °C with gentle shaking. After releasing cells from the tissue by continuous pipetting, residual tissue was removed by filtering the suspension through a 70-μm mesh filter. The filtered cell suspension was centrifuged at 290 g , and cells were washed in 5 ml HBSS+0.5% bovine serum albumin (HBSS/BSA). Cells were then resuspended in 800 μl HBSS/BSA and 25 μl (4×10 5 beads per μl) Dynabeads M-450 (Sheep anti-rat IgG, Invitrogen) coated with 1.5 μg anti-mouse CD144 antibody produced in rat (BD Pharmingen). Cells were incubated in an end-over-end shaker at room temperature for 30 min and unbound cells were removed by washing five times with HBSS/BSA, using a magnetic device (Dynal MPC-1, Invitrogen). Cells were plated onto fibronectin-coated cell culture dishes, cultured in endothelial cell growth medium (C-22020, Promocell, Heidelberg, Germany) supplemented with 15% fetal calf serum (PAA, Cölbe, Germany) and allowed to grow to confluency for 7–10 days. Cells were washed with HBSS/BSA and further purified by adding CD144-coated Dynabeads M-450 in HBSS/BSA, directly to the cell culture dish for 60 min. After trypsinization, unbound cells were removed by washing with HBSS/BSA, using the magnetic device as described above. The identity of endothelial cells was confirmed by staining with an antibody directed against von-Willebrand factor (number 1284924, Boehringer Mannheim, Mannheim, Germany) and platelet endothelial cell adhesion molecule-1 (M20 SC-1506, Santa Cruz Biotechnology, Santa Cruz, USA). An immunoblot with a TRPC6-specific antiserum (gift of V. Flockerzi) demonstrated the absence of the TRPC6 protein in endothelial cells of TRPC6-deficient mice. Determination of intracellular H 2 O 2 in MLEC For intracellular H 2 O 2 detection, the coding information for the H 2 O 2 -sensitive, enhanced yellow fluorescent protein variant HyPer [48] was subcloned under the control of the EF-1α enhancer/promoter into the pWPXL plasmid (distributed by Addgene, Boston) and packed with a second-generation lentivirus transduction system (see http://tronolab.epfl.ch/ for more details). Infections were carried out with a titre of at least 1×10 7 particles according to established protocols (see http://tronolab.epfl.ch/ for more details). The optimal HyPer signal-to-noise ratio was determined by acquiring continuous excitation–emission spectra in the presence or absence of 100-μM H 2 O 2 (data not shown). Experiments were carried out as outlined for the [Ca 2+ ] i -imaging and Mn 2+ -quench experiments in MLEC, but with 420 and 470 nm wavelength as excitation parameters. ESR spectroscopy measurements Superoxide generation in isolated lungs was measured by ESR spectroscopy, using the spin probe 1-hydroxy-3-carboxy-2,2,5,5-tetramethylpyrrolidine (CPH, Alexis Corporation, San Diego, CA, USA), as described [49] . Briefly, stock solutions of CPH (10 mmol l −1 ) dissolved in 0.9% NaCl that contained 1 mmol l −1 diethylenetriamine-pentaacetic acid, and was purged with argon, were prepared daily and kept under argon on ice. Diethylenetriamine-pentaacetic acid was used to decrease CPH autoxidation, which is catalysed by trace amounts of transition metals. Isolated mouse lungs were perfused with Krebs-HEPES buffer and then pretreated for 4 h with 50 g l −1 Chelex 100 to minimize transition metal contamination. Lungs from WT, Nox2 y/− or chimeric mice were exposed to anoxic ischaemia for 90 min. The spin probe, CPH (0.5 mmol l −1 ), was added into the perfusate 5 min before the onset of reperfusion. Samples from the venous outflow of the isolated lung were collected in 50-μl glass capillary tubes and measured immediately at room temperature. Samples were collected every 15 s during the first 3 min of reperfusion and then every 1 min or 5 min, as appropriate. Experiments were also carried out in time-matched non-ischaemic control lungs. The triple-line spectrum of 3-carboxy-proxyl radical (CP • ) was detected using an MS100 spectrometer (Magnettech, Berlin, Germany). The ESR settings were as follows: microwave frequency, 9.78 GHz; modulation frequency, 100 kHz; modulation amplitude, 2 G; microwave power, 18 mW. The quantity of trapped ROS was directly calculated from the change of the ESR signal intensity during the first 5 min of reperfusion. The superoxide portion of the ESR signal was calculated as the difference between the ROS release in the presence and absence of superoxide dismutase in buffer fluid (150 U ml −1 ). For the determination of superoxide generation by MLEC, cells were trypsinized and centrifuged at 320 g for 5 min. Supernatant was discarded and the sediment was resuspended and washed two times in ESR-Krebs HEPES buffer (Noxygen Science Transfer & Diagnostics GmbH, Germany). Samples were adjusted to cell numbers and incubated for 2 h at 37 °C. Incubation of parallel samples with superoxide dismutase (15 U ml −1 , Sigma-Aldrich, Germany) allowed calculation of the superoxide portion of the ESR signal. All samples were treated with CPH for 30 min at 37 °C. Measurements were performed using the Bruker EMX micro Spectrometer (Bruker Biospin, Steinheim, Germany). Electric cell impedance sensing (ECIS) Hypoxia-induced changes in endothelial resistance were analysed using an ECIS flow device (Applied Biophysics, Troy, USA). Impedance arrays (8F1E) were incubated with endothelial cell medium overnight. A total of 20,000 endothelial cells were seeded per well and grown for 48 h at 37 °C and 5% CO 2 in an incubator. Medium was removed, HBSS was added to the cells, and the array was connected to the ECIS device. HBSS was exchanged to HBSS gassed with N 2 as soon as impedance was stable. Resistance (Ω) was analysed for 3–5 h. How to cite this article: Weissmann, N. Activation of TRPC6 channels is essential for ischaemia–reperfusion-induced lung oedema in mice. Nat. Commun. 3:649 doi: 10.1038/ncomms1660 (2012).